Single-step deposition of high-mobility graphene at reduced temperatures Current methods of chemical vapour deposition (CVD) of graphene on copper are complicated by multiple processing steps and by high temperatures required in both preparing the copper and inducing subsequent film growth. Here we demonstrate a plasma-enhanced CVD chemistry that enables the entire process to take place in a single step, at reduced temperatures (<420 °C), and in a matter of minutes. Growth on copper foils is found to nucleate from arrays of well-aligned domains, and the ensuing films possess sub-nanometre smoothness, excellent crystalline quality, low strain, few defects and room-temperature electrical mobility up to (6.0±1.0) × 10 4 cm 2 V −1 s −1 , better than that of large, single-crystalline graphene derived from thermal CVD growth. These results indicate that elevated temperatures and crystalline substrates are not necessary for synthesizing high-quality graphene. Much progress has been made in growing large-area graphene by means of thermal chemical vapour deposition (CVD) based on catalytic dehydrogenation of carbon precursors on copper [1] , [2] , [3] , [4] . However, in many instances it is desirable to avoid multiple steps [2] and high temperatures ( ~ 1,000 °C) employed in thermal-CVD growth. In particular, the conditions for the critical removal of the native copper oxide and the subsequent film growth are dissimilar enough to necessitate separate process steps. Moreover, high processing temperatures restrict the types of devices and processes where CVD can be applied and can also result in film irregularities that compromise the graphene quality itself [4] . Thermally derived strain and topological defects, for example, can induce giant pseudo-magnetic fields and charging effects [5] , [6] , [7] , [8] , giving rise to localization and scattering of Dirac fermions [7] , [8] and diminishing the electrical properties. A variant of thermal CVD, called plasma-enhanced CVD (PECVD), has been widely used for depositing many allotropes of carbon, most notably diamond films. The plasma can provide a rich chemical environment, including a mixture of radicals, molecules and ions from a simple hydrogen-hydrocarbon feedstock [9] , allowing for lower deposition temperatures [10] and faster growth than thermal CVD. The ability of the plasma to support multiple reactive species concurrently is a key advantage. However, the quality of PECVD-grown graphene to date has not been significantly better than that of thermal CVD [10] , [11] , [12] . Here we demonstrate a PECVD process that encompasses both the preparation of the copper and growth of graphene in a single step. The addition of cyano radicals, which are known to etch copper at room temperature [13] , to a hydrogen-methane plasma is found to produce a chemistry whereby the native oxide is removed, the copper is smoothly etched, and growth of well-aligned graphene ensues. Etching of the copper substrate is found to be self-limiting, allowing etching and growth steps to proceed in tandem under the same chemistry. The entire process occurs in a matter of minutes without active heating, and the resulting graphene films exhibit high electrical mobility and few structural defects. Our results indicate that elevated temperatures, crystalline growth substrates, and long process times are not necessary for synthesizing high-quality graphene. Description and characterization of process The PECVD growth process is schematically illustrated in Fig. 1a–c and further described in Methods and Supplementary Fig. 1 . Copper was directly exposed to a low-pressure, microwave hydrogen plasma containing trace amounts of cyano radicals, methane and nitrogen ( Supplementary Fig. 2 and Supplementary Fig. 3 ), as detailed in Supplementary Note 1 . Removal of the native oxide and smoothing of the copper typically occurred within 2 min of igniting the plasma ( Fig. 1a ). Nucleation of graphene ensued on both sides of the substrate ( Fig. 1b ). With continued exposure to the plasma, disordered graphite and monolayer graphene covered the top and bottom sides, respectively ( Fig. 1c ). Copper deposits were found on both the process tube and the sample holder after successful growth runs ( Fig. 1d ), whereas runs with little copper etching did not produce optimal films. Optical microscopy showed that the top surface of the sample was always randomly pitted after growth ( Fig. 1e ), whereas that on the bottom surface was smooth ( Fig. 1f ). Scanning tunnelling microscopy (STM) measurements of the surface topography of graphene on the bottom side of Cu revealed sub-nanometre flatness for samples grown on Cu foils and single crystalline Cu (100) and Cu (111) ( Fig. 1g–i and Supplementary Fig. 5a–c ). Nitrogen incorporation into the graphene, as measured by X-ray photoemission spectroscopy, Supplementary Fig. 4a,b , was found to be below the detection limit [14] of 0.1 at.%. 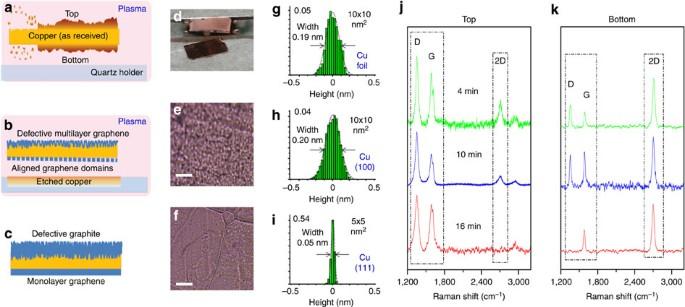Figure 1: PECVD-graphene growth process. (a) Exposure to plasma removes the native oxide and smoothes the copper substrate. (b) Aligned graphene nucleates on the bottom of the copper and disordered multilayer graphene forms on the top. (c) Monolayer graphene and disordered carbon develop on the bottom and top of the copper substrate, respectively, with continued exposure to plasma. (d) A copper foil and the sample holder, showing etched copper after PECVD growth. Optical images of the top (e) and bottom (f) of a copper foil after growth, where the scale bars correspond to 50 μm. (g) Height histogram for PECVD-graphene grown on Cu foil. (h) Height histogram for PECVD-graphene grown on single crystalline Cu (100). (i) Height histogram for PECVD-graphene grown on Cu (111). (j,k) Comparison of the time-evolved Raman spectra of the (j) top and (k) bottom of the Cu foil taken with increasing growth time. Figure 1: PECVD-graphene growth process. ( a ) Exposure to plasma removes the native oxide and smoothes the copper substrate. ( b ) Aligned graphene nucleates on the bottom of the copper and disordered multilayer graphene forms on the top. ( c ) Monolayer graphene and disordered carbon develop on the bottom and top of the copper substrate, respectively, with continued exposure to plasma. ( d ) A copper foil and the sample holder, showing etched copper after PECVD growth. Optical images of the top ( e ) and bottom ( f ) of a copper foil after growth, where the scale bars correspond to 50 μm. ( g ) Height histogram for PECVD-graphene grown on Cu foil. ( h ) Height histogram for PECVD-graphene grown on single crystalline Cu (100). ( i ) Height histogram for PECVD-graphene grown on Cu (111). ( j , k ) Comparison of the time-evolved Raman spectra of the ( j ) top and ( k ) bottom of the Cu foil taken with increasing growth time. Full size image We found that the occurrence of PECVD-graphene growth was largely insensitive to the gas temperature of the plasma. The maximum gas temperature of the plasma determined by a thermocouple sheathed in boron nitride was found to be 160 °C (425 °C) for 10 W (40 W) plasma power, which decayed by more than 120 °C (250 °C) within ~1 cm from the centre of the plasma. The maximum temperature of the copper substrate T s was measured using the melting points of known solids on top of a copper substrate subjected to the plasma. We found that at 40 W plasma power, lead melted whereas zinc did not, indicating that the maximum Cu substrate temperature was within the range of 327.5 °C< T s <419.5 °C. Further, we were able to fabricate more than 300 high-quality large-area graphene samples by PECVD within 5 – 20 min in a single-step by using plasma power varying between 10 and 40 W. The typical substrate size was (8 × 13) mm 2 . Although the plasma produced by the Evenson cavity was not uniform in intensity over the length of the sample, graphene was found to cover the entire substrate and exhibited consistent quality over the entire film on the bottom side, indicating that the growth was not temperature sensitive and could occur over a range of temperatures. We expect that the sample size should be scalable in a larger cavity under the same growth conditions. The localized nature of the plasma source also allowed multiple samples to be prepared individually in the same process tube without changing conditions or breaking vacuum by simply translating the Evenson cavity. Nucleation and growth The time evolution in the Raman spectra of PECVD-graphene on copper foils during growth is shown in Fig. 1j,k . Spectra from the top side ( Fig. 1j ) featured the D-band, an indicator of edges or disorder in graphene and graphite; the G-band, a feature common to both graphene and graphite; and the 2D-band, a feature that can be used to distinguish graphene from graphite [15] . The D-band was prominent throughout, whereas the 2D-band decreased and disappeared with time, indicating the formation of disordered graphite, which is consistent with optical images of the top side ( Fig. 1e ). In contrast, spectra from the bottom side ( Fig. 1k ) showed that the D-band decreased and eventually vanished with increasing growth time, whereas the relative intensities of 2D and G-bands indicate the formation of monolayer graphene [15] , [16] , [17] , [18] , as described in Methods and Supplementary Fig. 6a,b . This behaviour is consistent with growth and eventual coalescence of graphene domains wherein the D-band associated with the edge states of the domains diminished [19] . A comparison of the graphene from the top and bottom sides indicate that increased mass flux and direct plasma exposure adversely affected the film quality, and hereafter we focus our studies on PECVD-graphene grown on the bottom side of Cu. Scanning electron microscopy (SEM) images taken shortly after the onset of graphene growth on copper foil ( Fig. 2a–d ) revealed dense, linear arrays of hexagonal graphene domains that extended across the copper grains. With increasing growth time, the well-aligned graphene domains coalesced seamlessly into a monolayer graphene with few defects. Shown in Fig. 2e,f are the 2D/G and D/G intensity ratio maps of a (100 × 100) μm 2 area of an as-deposited graphene sample on Cu, respectively. The average 2D/G intensity ratio ( I 2D / I G ) is ~2 and only 5% of the mapped area show any measurable D-band. Histograms of the ( I 2D / I G ) and ( I D / I G ) maps are provided in Supplementary Fig. 6a,b , respectively. 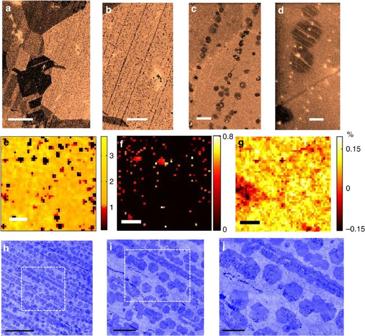Figure 2: Large-area characterization of PECVD-graphene on Cu. (a–d) False-colour SEM images of early-stage growth (with increasing magnification from left to right, where the scale bars correspond to 30 μm, 10 μm, 1 μm and 200 nm, respectively), showing extended linear arrays of well-aligned hexagonal domains (dark) on copper foil (light). (e) (100 × 100) μm2map (scale bar, 20 μm) of the Raman spectral 2D/G intensity ratio of a fully developed monolayer graphene sample on copper foil. (f) (100 × 100) μm2map (scale bar: 20 μm) of the Raman spectral D/G intensity ratio over the same area as ine; (g) (100 × 100) μm2strain map (scale bar, 20 μm) over the same area as ineandf. (h–j) False-colour SEM images of graphene grown for excessive time and transferred to single crystalline sapphire (with increasing magnification from left to right, where the scale bars corresponding to 30, 10 and 5 μm, respectively), showing well-aligned adlayer graphene domains (dark) on the bottom monolayer graphene (light). Figure 2: Large-area characterization of PECVD-graphene on Cu. ( a – d ) False-colour SEM images of early-stage growth (with increasing magnification from left to right, where the scale bars correspond to 30 μm, 10 μm, 1 μm and 200 nm, respectively), showing extended linear arrays of well-aligned hexagonal domains (dark) on copper foil (light). ( e ) (100 × 100) μm 2 map (scale bar, 20 μm) of the Raman spectral 2D/G intensity ratio of a fully developed monolayer graphene sample on copper foil. ( f ) (100 × 100) μm 2 map (scale bar: 20 μm) of the Raman spectral D/G intensity ratio over the same area as in e ; ( g ) (100 × 100) μm 2 strain map (scale bar, 20 μm) over the same area as in e and f . ( h – j ) False-colour SEM images of graphene grown for excessive time and transferred to single crystalline sapphire (with increasing magnification from left to right, where the scale bars corresponding to 30, 10 and 5 μm, respectively), showing well-aligned adlayer graphene domains (dark) on the bottom monolayer graphene (light). Full size image Although the number of graphene layers may be determined from the full-width half-maximum (FWHM) of the 2D-band [20] , the absolute value of the FWHM can be affected by the underlying substrate [21] . To avoid such complications, Raman maps of PECVD-graphene transferred from Cu to Si/SiO 2 are provided in Supplementary Fig. 7a–d and detailed in Methods and Supplementary Note 2 . The average value of the FWHM of the 2D-band, which was fit to a single Lorentzian, was 28.8 cm −1 , and the average ratio ( I 2D / I G )=2.7, both consistent with the figure of merit for monolayer graphene [15] , [16] , [17] , [18] , [20] . High-resolution (~1 nm) atomic force microscopy and SEM studies over multiple (100 × 100) μm 2 areas of an annealed monolayer graphene sample [22] , which was transferred to single crystalline sapphire with a polymer-free technique [23] , indicated no discernible grain boundaries. With an increase of growth time, small adlayers began to develop on top of the first layer in an aligned manner, as exemplified by the SEM images in Fig. 2h–j . These findings, which are supported by Fig. 1k , indicate that the growth of PECVD-graphene on copper foils proceeded by nucleation and growth of well-aligned domains [24] , [25] that eventually coalesced into a large single crystalline sheet, and the subsequent growth of the second layer with increasing time followed a similar mechanism ( Fig. 2h–j ). Strain and structural ordering The biaxial strain ( ε ll + ε tt ) in the PECVD-graphene on Cu can be estimated by considering the Raman frequency shifts and the Grneisen parameter [15] , [26] : where m (=G, 2D) refers to the specific Raman mode. Using the parameter , the strain distribution over an area of (100 × 100) μm 2 is exemplified in Fig. 2g , showing consistently low strain characteristics, with an average strain ~0.07% for m=2D. Overall, a general trend of downshifted G-band and 2D-band [15] was found for all PECVD-graphene relative to thermal CVD-grown graphene on the same substrate, as exemplified in Supplementary Fig. 8a–c for comparison of PECVD- and as-grown thermal CVD-graphene on substrates of Cu foil, Cu (100) and Cu (111). The consistent frequency downshifts for all PECVD-graphene indicate reduction in the averaged biaxial strain. Further, the absence of the D-band in most spectra suggests that the samples were largely free of disorder/edges on the macroscopic scale, which is further corroborated by detailed spatial mapping of the Raman spectra over an area of (100 × 100) μm 2 in Fig. 2e,f . The PECVD-graphene exhibited a well-ordered honeycomb atomic lattice, which is unique to monolayer graphene, as evidenced by the STM images of samples on Cu foil ( Fig. 3a–c ), Cu (100) ( Fig. 3e–g ) and Cu (111) ( Fig. 3i–k ). The long-range structural ordering was further corroborated by the sharp Fourier transformation (FT) of STM topographies, as exemplified in Fig. 3d,h,l . The FT spectra demonstrated dominantly hexagonal lattices for all PECVD-graphene. Samples grown on Cu single crystals further exhibited Moiré patterns, as manifested by the second set of smaller Bragg diffraction peaks. Simulations (see Methods) indicated the Moiré pattern (a parallelogram) in the FT of Fig. 3h for graphene on Cu (100), was the result of a square lattice at approximately an angle ~(12±2)° relative to the honeycomb lattice ( Supplementary Fig. 9a ), whereas the Moiré pattern (a smaller hexagon) in the FT of Fig. 3l suggested that the Cu (111) hexagonal lattice was at ~6±2° relative to the graphene lattice ( Supplementary Fig. 9b ). These STM measurement over multiple samples and multiple areas per sample confirm the predominance of monolayer graphene and the absence of discernible bilayer graphene in our PECVD-grown samples. 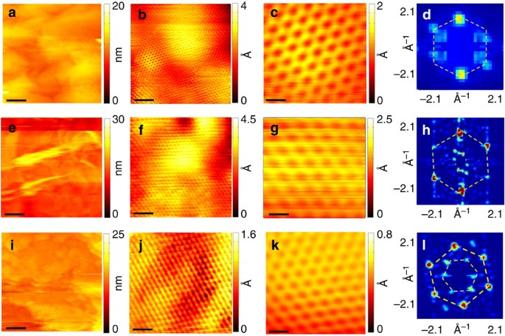Figure 3: Topographies of PECVD-graphene on copper. STM topographies of PECVD graphene at 77 K over successively decreasing areas (first three columns) and the corresponding Fourier transformation (FT) of large-area topography (fourth column) for samples grown on (a–d) Cu foil; (e–h) Cu (100); and (i–l) Cu (111). The scale bars fora,eandiare 40 nm; forb,fandjare 2 nm; and forc,gandkare 0.4 nm. Figure 3: Topographies of PECVD-graphene on copper. STM topographies of PECVD graphene at 77 K over successively decreasing areas (first three columns) and the corresponding Fourier transformation (FT) of large-area topography (fourth column) for samples grown on ( a – d ) Cu foil; ( e – h ) Cu (100); and ( i – l ) Cu (111). The scale bars for a , e and i are 40 nm; for b , f and j are 2 nm; and for c , g and k are 0.4 nm. Full size image The STM topography was further employed to analyse strain at the microscopic scale. For a local two-dimensional displacement field , where r and r 0 denote the actual position of a carbon atom and its equilibrium position in ideal graphene, respectively [27] , the compression/dilation strain is given by (∂ u x /∂ x )+(∂ u y /∂ y )≡ u xx + u yy , which is proportional to the biaxial strain [5] , [7] , [8] . Using the topographies shown in Fig. 3a–c , we obtained the spatial strain maps for PECVD-graphene on Cu foil, Cu (100) and Cu (111) substrates over successively decreasing areas in Fig. 4a,b,e ,f,i,j, respectively. The corresponding strain histograms are given in Fig. 4c,g,k . The PECVD-graphene exhibited low and relatively homogeneous strain distributions. Further comparison with the macroscopic strain obtained from a collection of Raman spectra taken on different areas of multiple PECVD-graphene samples are summarized by the strain histograms in Fig. 4d,h,l . There is overall consistency between microscopic STM studies and macroscopic Raman spectroscopic studies, revealing low strain for all PECVD-graphene. 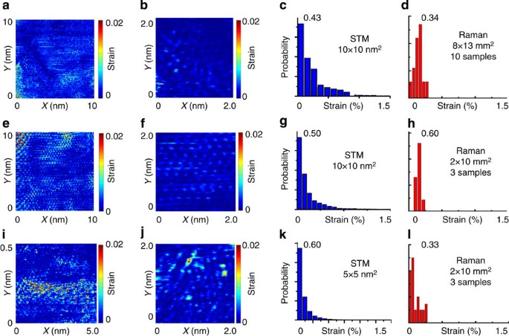Figure 4: Comparison of the spatially resolved strain maps and strain histograms of PECVD-graphene. From left to right, compression/dilation strain maps over successively decreasing areas taken with STM at 77 K (first and second columns, colour scale in units of %), strain histogram (third column) of the strain map shown in the first column, and strain histogram (fourth column) obtained from Raman spectroscopic studies of different areas of multiple PECVD-graphene samples grown on (a–d) Cu foil, (e–h) Cu (100) and (i–l) Cu (111). The strain obtained from STM topography is largely consistent with the findings from Raman spectroscopic studies. Figure 4: Comparison of the spatially resolved strain maps and strain histograms of PECVD-graphene. From left to right, compression/dilation strain maps over successively decreasing areas taken with STM at 77 K (first and second columns, colour scale in units of %), strain histogram (third column) of the strain map shown in the first column, and strain histogram (fourth column) obtained from Raman spectroscopic studies of different areas of multiple PECVD-graphene samples grown on ( a – d ) Cu foil, ( e – h ) Cu (100) and ( i – l ) Cu (111). The strain obtained from STM topography is largely consistent with the findings from Raman spectroscopic studies. Full size image Electrical properties The electrical mobility ( μ ) of PECVD-graphene was determined by studying back-gated field-effect-transistor devices [28] , [29] . Graphene samples were first transferred to hexagonal boron nitride (BN) thin films on 300 nm SiO 2 /Si substrates using a polymer-free method [23] , and then lithographically processed into a geometry shown in Fig. 5a,b . The sheet resistance of graphene as a function of the back-gate voltage ( V ) and the corresponding conductivity ( σ ) versus sheet carrier density ( n s ) were measured at 300 K, as exemplified in Fig. 5c,d . 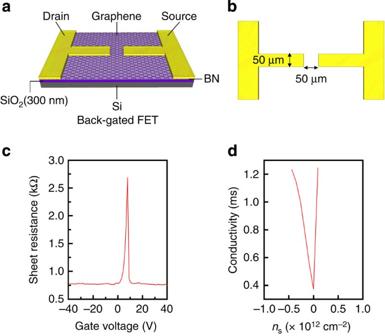Figure 5: Electrical mobility measurements. (a) Schematics of a typical back-gated field-effect-transistor (FET) device and (b) detailed dimensions of the top view. (c) Representative sheet resistance versus gate voltage (V) data taken at 300 K for PECVD-graphene on Cu foil and transferred to BN. (d) Conductivity (σ) versus sheet carrier density (ns) data converted froma. A set of electron mobility (μ) data from nine different FET devices based on PECVD-graphene grown on Cu foils are summarized inTable 1, whereμ=(1/C) (dσ/dV) was determined at the charge neutrality point. The errors for each device due to discreteness of the voltage readings exemplified incare within ±15% of the tabulated mean value. The electrical mobility μ was obtained from the derivative of the Drude formula [28] near the charge neutrality point: Figure 5: Electrical mobility measurements. ( a ) Schematics of a typical back-gated field-effect-transistor (FET) device and ( b ) detailed dimensions of the top view. ( c ) Representative sheet resistance versus gate voltage ( V ) data taken at 300 K for PECVD-graphene on Cu foil and transferred to BN. ( d ) Conductivity ( σ ) versus sheet carrier density ( n s ) data converted from a . A set of electron mobility ( μ ) data from nine different FET devices based on PECVD-graphene grown on Cu foils are summarized in Table 1 , where μ =(1/ C ) (d σ /d V ) was determined at the charge neutrality point. The errors for each device due to discreteness of the voltage readings exemplified in c are within ±15% of the tabulated mean value. Full size image where C denotes the capacitance of the device. The electrical mobility obtained from nine different devices was found to range from (3.0±0.5) × 10 4 to (6.0±1.0) × 10 4 cm 2 V −1 s −1 for electrons, as summarized in Table 1 , and from (1.2±0.2) × 10 4 to (3.5±0.5) × 10 4 cm 2 V −1 s −1 for holes, where the errors represented variations in determining the (d σ /d V ) slope due to the discreteness of voltage readings. These values are comparable to those obtained on large, single crystalline thermal CVD-grown graphene on BN, the latter yielded μ =4 × 10 4 to 6 × 10 4 cm 2 V −1 s −1 at 1.7 K and ~1.5 × 10 4 to 3 × 10 4 cm 2 V −1 s −1 at 300 K (ref. 2 ). Table 1 Electron mobility ( μ ) data from nine different FET devices based on PECVD-graphene. Full size table It is worth commenting on the accuracy of mobility values obtained by the two-terminal configuration depicted in Fig. 5a,b . The contact resistance between electrode and graphene was determined by the Transmission Line Model method and was found to be typically ~10 Ω for all devices. In contrast, the sheet resistance of graphene was typically more than 1 kΩ near the charge neutrality point, which was about two orders of magnitude larger than the contact resistance. Therefore, the contact resistance would not affect the accuracy of the mobility significantly. Additional measurements by patterning some of the PECVD-graphene into the four-point configuration revealed that the differences in mobility thus determined was less than 2–3% from those obtained by means of the two-point method. Experience with diamond PECVD lends understanding to the observed nucleation and growth of aligned graphene domains presented here. In the case of diamond growth, it is known to involve a competition between growth by carbon radicals (most notably methyl radicals) and etching of amorphous or disordered carbon by atomic hydrogen. The process conditions used in our experiments are similar to those of microwave CVD growth of diamond thin films. Therefore, it is not unreasonable to expect that our PECVD growth of graphene also proceeds in a competitive manner [30] . Further, diamond is known to nucleate preferentially via surface defects [31] , [32] , and the aligned domains in our work were found to be commensurate with the inherent machine marks on the as-received copper foils. Although the copper surface is smoothed during the PECVD process, remnants of the defects are likely because the process temperature is low. For comparison, aligned nucleation was not observed on single-crystal copper, which contains no marks. For thermal CVD growth of large, single-crystal graphene [2] , it is preferable to have smooth, defect-free substrates and restricted nucleation. Therefore, multiple steps to prepare the substrates before thermal CVD growth and post annealing after the growth to optimize the sample are necessary [2] . In contrast, graphene with equivalent or even better mobility can be achieved by the one-step PECVD process described in this work. This PECVD process is also scalable [11] , occurs at CMOS compatible temperatures, and avoids complications with multiple steps and post-processing. Overall, our findings of the guided PECVD growth process not only shed new light on the growth kinetics of graphene but also open up a new pathway to large-scale, excellent quality and fast graphene fabrication. In particular, this one-step PECVD process potentially allows graphene to be used as-deposited, making it amenable for integration with complementary materials and technology. Experimental setup The experimental setup is summarized in Supplementary Fig. 1 , which consists of plasma, vacuum and gas delivery systems. The plasma system (Opthos Instruments Inc.) consists of an Evenson cavity and a power supply (MPG-4), which provides an exciting frequency of 2,450 MHz. The Evenson cavity mates with a quartz tube of inner and outer diameters of 10 and 12.5 mm, respectively. The vacuum system is comprised of a mechanical roughing pump, two capacitance manometers, a pressure control valve and a measurement control system. There is a fore-line trap between the vacuum pump and the MKS 153 control valve. The gas delivery system consists of mass flow controllers (MFCs) for H 2 , CH 4 and Ar. A bakeable variable leak valve is placed before the methane MFC, and there is a leak valve for N 2 . A gas purifier was placed before the variable leak valve on the methane line. Quarter-turn, shut-off valves are placed directly after each of the MFCs. The system pressure and gas flows are monitored and controlled through the controller via a LabView interface. A residual gas analyzer (RGA) is used to monitor the exhaust gas. Detailed PECVD growth procedure and information The copper substrates were placed on a quartz flat inside of quartz tube. A typical substrate size was (8 × 13) mm 2 . The tube was evacuated to 25–30 mTorr. A 2–5 standard-cubic-centimeters-per-minute (s.c.c.m.) flow of room temperature hydrogen gas with 0.4% methane and a comparable amount of nitrogen gas was added and the pressure was controlled at 500 mTorr. The addition of methane to the gas flow was controlled by a precision leak valve, and a typical concentration, as measured by gas chromatography, was 0.4%. The initially low vacuum conditions (~25 mTorr) provided sufficient partial pressures of nitrogen (atmospheric) for the PECVD process. (We note that a leak valve for including purified nitrogen was added to the setup to study the effects of increased nitrogen partial pressures.) Typical partial pressures measured by RGA are as follows: N 2 (Mass 28): 6.9 × 10 −8 Torr CH 4 (Mass 16): 1.5 × 10 −7 Torr O 2 (Mass 32): 5.4 × 10 −9 Torr H 2 O (Mass 18): 1.2 × 10 −6 Torr CO 2 (Mass 44): 2.3 × 10 −8 Torr From these values, we estimate that the concentration of nitrogen in the gas flow is typically on the same order as that of methane. The PECVD process was found to be highly sensitive to the relative amounts of methane and nitrogen. Excessive methane mixtures resulted in no etching, whereas excessive nitrogen mixtures would result in excessive etching of the copper. Slight adjustments to the methane concentration could be made via either optical emission spectroscopy or RGA. A low-power (ranging from 10 to 40 W) cold hydrogen plasma was formed over the copper substrate using an Evenson cavity. Exposure of copper substrates to the plasma enabled continuing etching and cleansing of the copper surface during the graphene growth process. The gas temperature inside the plasma was measured using a thermocouple sheathed in boron nitride. The thermocouple was placed in the plasma above the sample and could be translated along the tube. The peak gas temperature measured in plasma treatment was 160 °C at 10 W and 425 °C at 40 W, and the gas temperature profile decreased rapidly (by 120 °C at 10 W and 425 °C at 40 W within 1 cm) from the peak value. The maximum temperature of the copper substrate T s was measured using the melting point of known solids, lead and zinc, and found to be within the range of 327.5 °C< T s <419.5 °C at 40 W. Typically after 5–20 min of direct exposure to the plasma, a large-area monolayer graphene formed on the backside of copper substrates, whereas the front side of the substrates was coated with disordered graphite. Upon the completion of graphene growth, the plasma was extinguished, and the gas flows were stopped. The process tube was then evacuated and back filled with Ar, and the substrate with graphene coating was subsequently removed. Copper deposition was visible on the inside of the tube and on the sample holder as the result of plasma etching of the copper substrates. Analysis of monolayer graphene using Raman spectroscopy The Raman maps shown in Fig. 2e,f of the manuscript for PECVD-graphene on Cu were collected with Renishaw InVia @ 532 nm, and the spectra were taken at 2 μm per pixel steps over an area of (100 × 100) μm 2 for a total of 2,601 spectra. Similarly, the Raman maps in Supplementary Fig. 7a,b for PECVD-graphene transferred to SiO 2 were taken at 2 μm per pixel steps over an area of (160 × 150) μm 2 . Each spectrum was smoothed and the broad background from the copper fluorescence was removed, and the peak locations and intensities for the D, G and 2D features were extracted. The relative intensities of the 2D and G-band and those of the D and G-band are presented in Fig. 2e,f , and histograms of the ratio values and the FWHM linewidth of the 2D band of our PECVD-grown graphene on Cu and commercial thermal CVD-grown graphene on Cu are shown in Supplementary Fig. 6a–e . The predominant ( I D / I G )~0 value of the graphene sample shown in Supplementary Fig. 6a indicates negligible defects, whereas the histogram of the 2D/G intensity ratio ( I 2D / I G ) shown in Supplementary Fig. 6b reveals that the average of the ( I 2D / I G ) value is ~2, which agrees with the figure of merit ( I 2D / I G )>1 for monolayer graphene [15] , [16] , [17] , [18] . This notion of predominantly monolayer graphene described in this work is further corroborated by detailed studies of a PECVD-graphene sample transferred from Cu to a SiO 2 substrate, which prevents the complication of slow oxidation of the Cu substrate that could result in the 2D linewidth broadening with time due to the influence of the substrate (see Supplementary Note 2 ). As shown in Supplementary Fig. 7a–d , a large spatial map over an area of (160 × 150) μm 2 revealed a mean FWHM value=28.8 cm −1 for the 2D-band and a mean value ( I 2D / I G )=2.7, both are consistent with predominantly monolayer graphene if we use either the criterion of 2D-band FWHM<30 cm −1 as the figure of merit for monolayer graphene on SiO 2 (ref. 20 ) or the criterion ( I 2D / I G )>1 for monolayer graphene on various substrates [15] , [16] , [17] , [18] . Simulations Simulations of the Moiré patterns and the corresponding FT were made by means of Matlab. We generated the triangular and cube lattices by using cosine square function and the hexagonal lattice by displacement of two triangular lattice functions. The lattice constant for the ideal 2D honeycomb structure of graphene is 0.2461, nm and that for the ideal Cu FCC lattice is 0.3615, nm, which has a corresponding lattice constant for the triangular lattice in the 111 direction and the square lattice in the 100 direction. To simulate realistic STM imaging of the Moiré pattern for a given relative angle θ between the top graphene layer and the underlying Cu lattice, we assume the resulted topological function G ( x , y ) has the following form: where 0< r ≤1, G C ( x , y ) is the graphene honeycomb lattice function and G Cu ( x , y , θ ) is the copper layer function which could be either the triangular lattice for Cu (111) or the cubic lattice for Cu (100). Both functions are normalized with maximum 1 and minimum 0. We use the exponent in equation (3) to simulate the rapid decay of the tunnelling current contribution from the copper atom directly under a carbon atom in the top graphene layer, where k is a parameter that controls the decay rate and was chosen to be 2–4. Even for exposed copper atoms without any carbon atom directly positioning above, the signal from copper is expected to be attenuated by a ratio r due to a larger distance from the STM tip to the copper layer. The above expression ensures that contributions from copper atoms directly under carbon atoms are much reduced due to deflection of tunnelling electrons, whereas those from exposed copper atoms are only attenuated by a coefficient r . The matching between simulations and the Fourier transform (FT) of graphene on Cu (100) lattice data is judged by the angle of inner parallelism. At θ =(12±2)°, the angle of the inner parallelism appear to match the experimental result in Fig. 3h , as shown in by the real space Moiré pattern (left panel) and the corresponding FT (right panel) in Supplementary Fig. 9a . In contrast, the matching between simulations and the FT of graphene on Cu (111) data is based on the size of inner hexagon relative to that of the outer hexagon for the graphene lattice. In fact, there are actually two inner hexagons according to the simulations, as exemplified in the FT of the Moiré pattern in Supplementary Fig. 9b for θ =(6±2)°. However, empirically only the larger inner hexagon is visible ( Fig. 3l ). We attribute this discrepancy to the intense DC signal from the zone centre of the FT spectra, which overwhelms the signal of the smaller inner hexagon and so becomes invisible upon our removal of the DC signal. How to cite this article: Boyd, D. A. et al. Single-step deposition of high-mobility graphene at reduced temperatures. Nat. Commun. 6:6620 doi: 10.1038/ncomms7620 (2015).